Three functionally distinct classes of C-fibre nociceptors in primates In primates, C-fibre polymodal nociceptors are broadly classified into two groups based on mechanosensitivity. Here we demonstrate that mechanically sensitive polymodal nociceptors that respond either quickly (QC) or slowly (SC) to a heat stimulus differ in responses to a mild burn, heat sensitization, conductive properties and chemosensitivity. Superficially applied capsaicin and intradermal injection of β-alanine, an MrgprD agonist, excite vigorously all QCs. Only 40% of SCs respond to β-alanine, and their response is only half that of QCs. Mechanically insensitive C-fibres (C-MIAs) are β-alanine insensitive but vigorously respond to capsaicin and histamine with distinct discharge patterns. Calcium imaging reveals that β-alanine and histamine activate distinct populations of capsaicin-responsive neurons in primate dorsal root ganglion. We suggest that histamine itch and capsaicin pain are peripherally encoded in C-MIAs, and that primate polymodal nociceptive afferents form three functionally distinct subpopulations with β-alanine responsive QC fibres likely corresponding to murine MrgprD-expressing, non-peptidergic nociceptive afferents. Unmyelinated nociceptive afferents in primate are classified primarily based on their receptive properties as either polymodal afferents sensitive to mechanical, thermal and chemical stimuli (CMH) or mechanoinsensitive (C-MIA) afferents. CMH fibres have been studied extensively across different species and are the most common nociceptor type encountered in recordings from peripheral nerves [1] , [2] , [3] , [4] , [5] . Psychophysical and electrophysiological studies suggest that CMHs encode pain sensation induced by noxious heat stimuli [6] , [7] and are involved in mediating non-histaminergic itch from cowhage spicules [8] , [9] . In primate, CMHs respond to intradermal injection of histamine [8] , but their role in histamine-induced itch is still unclear. Intradermal capsaicin injection does not lead to a sustained activation in these afferents [8] , [10] , [11] , although capsaicin desensitization of human skin, paradoxically, leads to loss of cowhage-induced itch [12] and heat sensation [13] . Primate CMHs exhibit either a quick (QC) or slow (SC) response to a stepped heat stimulus [8] , [14] . The basis for this dichotomy is unknown. One possibility is that the terminals of QCs are located more superficially in the skin than those of SCs. An alternative hypothesis, supported by the data presented in this manuscript, is that QCs and SCs represent two distinct populations of polymodal nociceptors. In mice, nociceptive dorsal root ganglion (DRG) neurons express a family of G protein-coupled receptors related to Mas-1 (Mrgprs), with different Mrgprs being expressed in distinct, non-overlapping neuronal subpopulations [15] . In electrophysiological recordings, CMHs were observed in the MrgprD- and MrgprA3 subpopulation [16] , [17] . MrgprD neurons are involved in nocifensive behaviour to mechanical stimuli [18] , [19] and in β-alanine-induced itch sensation [16] , whereas MrgprA3 neurons likely constitute a specific line for itch [17] , [20] . In primate, orthologous genes for some Mrgprs exist ( MrgD-G ) and genes that cannot be clearly assigned to any of the MrgA-C subfamilies described in mice ( MrgX1-4 ) [15] , [21] . However, the functional properties of Mrgpr-expressing neurons in primate that may correspond to neuronal subclasses described in mice are currently unknown. One aim of the present studies was to test whether QC- and SC afferents in primate represent distinct neuronal populations by investigating their receptive and conductive properties, including their responses to different chemical stimuli. Compared with CMHs, mechanically insensitive C-fibre afferents (C-MIAs) show a sustained activation following intradermal injections of histamine and capsaicin, and C-MIAs are therefore thought to play a crucial role in mediating itch and pain [11] , [22] . How histamine itch and capsaicin pain are encoded by activity in a single class of afferents is not well understood. Our findings indicate that primate polymodal nociceptors consist of three major subpopulations. Two are mechanoheat sensitive but have distinct physiological properties and sensitivity to β-alanine. The third subpopulation (C-MIAs) is unresponsive to mechanical stimuli and to β-alanine but exhibits distinct discharge patterns in response to intradermal injection of histamine and capsaicin. We conclude that β-alanine responsive QC fibres correspond to murine MrgprD expressing, non-peptidergic nociceptive afferents and that a peripheral coding mechanism in C-MIAs accounts for histamine itch and capsaicin pain. Polymodal C nociceptors exhibit two types of heat response CMHs exhibit two types of responses to a stepped heat stimulus (49 °C for 3 s, Fig. 1a ). One type ( Fig. 1b , red circles) is characterized by a burst of activity at the onset of the response. The second type ( Fig. 1b , blue circles) is characterized by a low frequency, sustained discharge throughout the stimulation period. 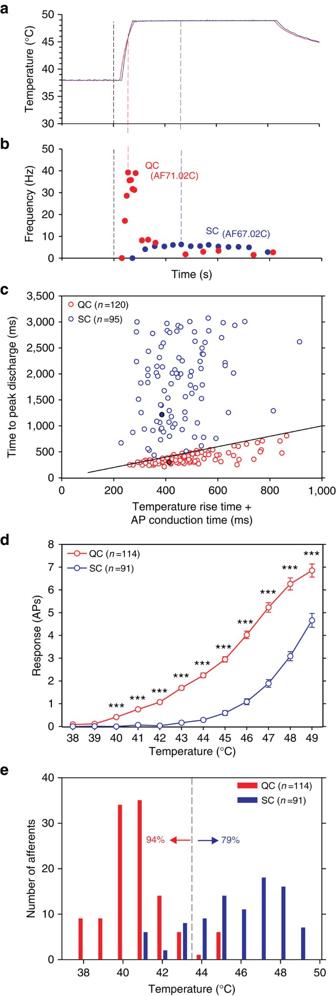Figure 1: The response to a 49 °C, 3-s stepped heat stimulus separates two classes of mechanoheat sensitive C fibres. (a) Temperature waveforms of the heat stimulus. The skin was first heated to a 38 °C, 3 s baseline temperature and then stepped (rise time<500 ms) to a 49 °C, 3-s. stimulus. The starting time of the temperature waveform was shifted by the conduction latency of each fibre to align it with the fibre’s response. (b) Specimen recording showing the response of a QC fibre (red circles) and an SC fibre (blue circles) to the stimulus depicted ina. Instantaneous discharge frequency is plotted versus time with each dot representing an action potential. In QC fibres, the evoked response starts during the rise in temperature, shows an early high frequency discharge (as indicated by the red dashed line), but quickly adapts during the stimulus duration. In contrast, the response of SC fibres reaches a peak during the plateau phase of the stimulus (as indicated by the blue dashed line). Start of the stimulus is indicated by the black dashed line. (c) The time of peak discharge for each fibre is plotted as a function of the stimulus rise time plus the conduction time for that fibre. Data points below the line of equality (solid line) correspond to those fibres whose peak discharge occurred during the rising phase of the heat stimulus. The two highlighted symbols show the data points for the examples AF71.02C and AF67.02C whose responses were plotted inbandSupplementary Fig. 2. (d) Average response to heat staircase stimulus (36 or 38–49 °C in 1 °C, 1-s increments) for SC and QC fibres. Mean number of APs (±s.e.m.) recorded at a given temperature was plotted against applied temperature. Responses at given temperatures were compared between QC and SC fibres using Mann–WhitneyU-test (***P<0.001). (e) Histogram of heat thresholds for QC and SC fibres. No QC had a heat threshold greater than 45 °C, whereas no SC had a heat threshold less than 41 °C. All data were collected in cynomolgus monkeys. Figure 1: The response to a 49 °C, 3-s stepped heat stimulus separates two classes of mechanoheat sensitive C fibres. ( a ) Temperature waveforms of the heat stimulus. The skin was first heated to a 38 °C, 3 s baseline temperature and then stepped (rise time<500 ms) to a 49 °C, 3-s. stimulus. The starting time of the temperature waveform was shifted by the conduction latency of each fibre to align it with the fibre’s response. ( b ) Specimen recording showing the response of a QC fibre (red circles) and an SC fibre (blue circles) to the stimulus depicted in a . Instantaneous discharge frequency is plotted versus time with each dot representing an action potential. In QC fibres, the evoked response starts during the rise in temperature, shows an early high frequency discharge (as indicated by the red dashed line), but quickly adapts during the stimulus duration. In contrast, the response of SC fibres reaches a peak during the plateau phase of the stimulus (as indicated by the blue dashed line). Start of the stimulus is indicated by the black dashed line. ( c ) The time of peak discharge for each fibre is plotted as a function of the stimulus rise time plus the conduction time for that fibre. Data points below the line of equality (solid line) correspond to those fibres whose peak discharge occurred during the rising phase of the heat stimulus. The two highlighted symbols show the data points for the examples AF71.02C and AF67.02C whose responses were plotted in b and Supplementary Fig. 2 . ( d ) Average response to heat staircase stimulus (36 or 38–49 °C in 1 °C, 1-s increments) for SC and QC fibres. Mean number of APs (±s.e.m.) recorded at a given temperature was plotted against applied temperature. Responses at given temperatures were compared between QC and SC fibres using Mann–Whitney U- test (*** P <0.001). ( e ) Histogram of heat thresholds for QC and SC fibres. No QC had a heat threshold greater than 45 °C, whereas no SC had a heat threshold less than 41 °C. All data were collected in cynomolgus monkeys. Full size image We sought a formal criterion to separate the two types. In a given afferent, the response profile to a stepped heat stimulus is influenced by several physical and physiological properties including: (1) the time needed to raise the temperature at the skin surface from baseline (38 °C) to the target temperature (49 °C) (that is, temperature rise time of 200–500 ms), (2) the time needed to raise the temperature at the depth of the receptive ending to the threshold temperature, (3) the time needed to initiate an action potential and (4) the time needed to conduct the action potential from the receptive ending to the recording electrode (that is, conduction time, ~\n100–300 ms). Among these variables, the temperature rise time and the conduction time are the largest contributors and, currently, the only measurable quantities. Therefore, the time of peak response frequency (relative to stimulus onset) was plotted against the sum of temperature rise time (as measured by the radiometer of our CO 2 laser system) plus the conduction latency of the afferent. The data points fell into two clusters ( Fig. 1c ): For about half of the afferents, data points fell on or below the line of equality (black line) indicating that the time to peak discharge was smaller than the sum of temperature rise time plus conduction latency of these afferents. The peak discharge in these afferents must have occurred during the rising phase of the temperature, and we therefore classify these afferents as ‘quick’ C fibres (QC, red circles). In contrast, data points for the remaining fibres were situated above the diagonal. In these ‘slow’ C fibres (SC, blue circles), the time of peak discharge exceeded the sum of temperature rise time and conduction latency. As shown in Fig. 1c , the ‘QC/SC’ classification was unambiguous for the vast majority of fibres, and only 1/95 SCs appears to fall onto the diagonal line. However, the observed peak instantaneous frequency in this afferent was that of a typical SC fibre, and therefore it was classified as such. Of 216 CMHs tested in cynomolgus monkeys, 121 (56%) were classified as QC, and 95 (44%) as SC. Peak discharge frequency and total number of action potentials (APs) evoked by the stepped heat stimulus were significantly larger in QCs than SCs ( Table 1 ). Both had positively accelerating stimulus response functions to an ascending heat staircase ( Fig. 1d ). The total response to the staircase was significantly larger in QCs than SCs ( Table 1 ). The percentage of cold sensitive polymodal C fibres was low (13/139), with the majority ( n =11) being QCs ( Table 1 ). Consistent with findings from microneurography recordings in humans [11] , a few C fibre afferents (3/219) were mechanosensitive only. Table 1 QCs and SCs have distinctly different properties Full size table The heat threshold of QCs was significantly lower than in SCs ( Table 1 ). The majority of the QCs (94%;107/114) had thresholds less than 44 °C ( Fig. 1e ) compared with only 21% of the SCs (16/91; P <0.001, χ 2 test). If QCs and SCs indeed represent distinct populations of nociceptive neurons, one would also expect to find such distinction in a different species. Similar to CMHs in cynomolgus monkeys, we found that CMHs in pigtail monkey could be differentiated into QCs and SCs (see Supplementary Fig. 1 ). As in cynomolgus monkeys, QCs in pigtail monkeys were more sensitive to mechanical and thermal stimuli than SCs (see Supplementary Table 1 ). In some properties (see Supplementary Table 1 ), QC and SC afferents in pigtail monkeys differed significantly from their counterparts in cynomolgus monkeys, and this may be due to species differences in skin properties (for example, thickness, softness). The mechanical thresholds of QCs were lower than in SCs ( Table 1 , Supplementary Table 1 ). Responses to the three suprathreshold von Frey hairs tested were larger in QCs than SCs ( Supplementary Fig. 2 , Table 1 ). In summary, these data indicate that QCs and SCs have distinctly different heat and mechanical response properties. The greater sensitivity of QCs could be explained by physical differences; for example, QCs may be located more superficially in the skin than the SCs. Alternatively, QCs and SCs may represent two molecularly distinct populations. To investigate this latter possibility, we studied the responses of QCs and SCs to other physiological stimuli. QCs and SCs sensitize differently after a mild burn injury We first investigated whether QCs and SCs in cynomolgus monkeys respond differently following a mild burn injury (48 °C, 2 min) that produced heat hyperalgesia in humans [23] . Before and after this burn, heat sensitivity was assessed with multiple heat staircases (37–49 °C in 1 °C, 1-s increments). Both fibre types became sensitized to heat (for typical examples, see Supplementary Fig. 3 ) as indicated by a leftward shift in their stimulus-response functions ( Fig. 2a,b ). However, SCs exhibited a greater sensitization, including a greater decrease in heat threshold and a greater increase in total evoked response to the heat staircase following the burn ( Table 1 , Supplementary Fig. 4 ). The sensitization was temperature dependent, and the curves showing the increase in response at a given temperature had unique shapes for each fibre type ( Fig. 2c ): QCs showed the biggest increase in the heat-evoked response at 45 °C whereas the response increase to 49 °C was smaller. In contrast, SCs sensitized over the whole temperature range with the largest increase in response at 49 °C. 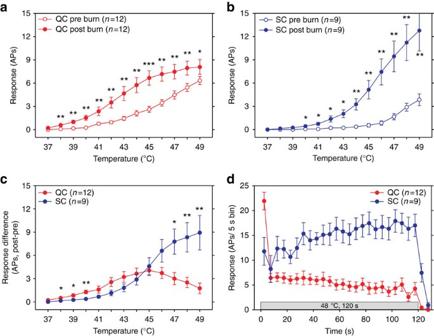Figure 2: SC afferents show greater sensitization to heat after a mild burn injury than QC afferents. (a,b) Averaged stimulus-response functions to the heat staircase before and after the mild burn injury. The increase in response after the burn for the QC afferents (a) reached a plateau at the higher stimulus temperatures. In contrast, the SC afferents (b) showed an enhanced response for all temperatures. Pre- and post-burn data were first analysed with Friedman analysis of variance (ANOVA) (pre QC:χ2(12,12)=138.2,P<0.001; post QC:χ2(12,12)=123.7,P<0.001; pre SC:χ2(9,12)=90.0,P<0.001; post SC:χ2(9,12)=101.3,P<0.001). Within each fibre class, pre- and post-burn data at a given temperature were compared with Wilcoxon matched pairs test (*P<0.05; **P<0.01; ***P<0.001) (c): The increase in heat response in QC and SC fibres is temperature dependent (QCs: Friedman ANOVAχ2(12,12)=81.6,P<0.001; SCs: Friedman ANOVAχ2(9,12)=99.1,P<0.001). In QCs, the largest change in response was observed at temperatures around 45 °C, whereas in SCs, the largest increase was observed at the higher temperatures. At low temperatures (37–39 °C) and high temperatures (47-49 °C), the change in response was significantly different between the groups (*P<0.05; **P<0.01; Mann–WhitneyU-test). (d): Time course of the averaged neuronal response of QC and SC fibres to the 48 °C, 120-s mild burn injury (bin size=5 s). The discharge in the QC afferents adapted quickly, whereas the average response of the SC afferents increased during the burn. Error bars indicate s.e.m. Data are exclusively from cynomolgus monkeys. Figure 2: SC afferents show greater sensitization to heat after a mild burn injury than QC afferents. ( a , b ) Averaged stimulus-response functions to the heat staircase before and after the mild burn injury. The increase in response after the burn for the QC afferents ( a ) reached a plateau at the higher stimulus temperatures. In contrast, the SC afferents ( b ) showed an enhanced response for all temperatures. Pre- and post-burn data were first analysed with Friedman analysis of variance (ANOVA) (pre QC: χ 2 (12,12) =138.2, P <0.001; post QC: χ 2 (12,12) =123.7, P <0.001; pre SC: χ 2 (9,12) =90.0, P <0.001; post SC: χ 2 (9,12) =101.3, P <0.001). Within each fibre class, pre- and post-burn data at a given temperature were compared with Wilcoxon matched pairs test (* P <0.05; ** P <0.01; *** P <0.001) ( c ): The increase in heat response in QC and SC fibres is temperature dependent (QCs: Friedman ANOVA χ 2 (12,12) =81.6, P <0.001; SCs: Friedman ANOVA χ 2 (9,12) =99.1, P <0.001). In QCs, the largest change in response was observed at temperatures around 45 °C, whereas in SCs, the largest increase was observed at the higher temperatures. At low temperatures (37–39 °C) and high temperatures (47-49 °C), the change in response was significantly different between the groups (* P <0.05; ** P <0.01; Mann–Whitney U- test). ( d ): Time course of the averaged neuronal response of QC and SC fibres to the 48 °C, 120-s mild burn injury (bin size=5 s). The discharge in the QC afferents adapted quickly, whereas the average response of the SC afferents increased during the burn. Error bars indicate s.e.m. Data are exclusively from cynomolgus monkeys. Full size image SCs also had a significantly greater response to the burn than QCs ( Fig. 2d , Table 1 ), which is the opposite of what was seen for the 49 °C, 3-s stimulus. This is because the QC response adapted quickly ( Fig. 2d ) such that the average response during the second 5-s period of the burn (6.4±0.8 APs) was significantly lower than in the first 5-s period (21.9±1.8 APs, P <0.001). In contrast, the response in SCs did not adapt during the burn ( Table 1 ). The QC/SC difference in the post-burn stimulus-response function, the difference in temperature-dependent sensitization and the difference in the burn response cannot be explained by the receptive terminals of QCs being located more superficially than SCs. Other intrinsic factors (for example, heat transduction mechanisms, second messenger systems) must exist that account for these differences. QCs and SCs differ in conduction properties To investigate whether QCs and SCs differ in conduction slowing properties, fibres were stimulated with suprathreshold electrical stimuli in the vicinity of their peripheral receptive fields (RF). Electrical stimulation bypasses the receptive terminals and directly activates the axon. Thus, the effects of electrical stimulation are independent of the depth at which receptive terminals are located within the skin. The latency of QCs and SCs increased (that is, the conduction velocity decreased) throughout the 3 min of stimulation at 2 Hz ( Supplementary Fig. 5 ). To combine data across fibres, we computed the change in conduction velocity during the electrical stimulation ( Fig. 3 , Supplementary Fig. 5C ). Data from pigtail and cynomolgus monkeys were combined as slowing did not differ between species (see Table 1 ). We also included in this analysis 9 C-MIAs tested with the same stimulation protocol. Overall slowing and slowing over the course of the stimulation differed significantly between fibre classes ( Fig. 3 ). At the end of the stimulation, the decrease in conduction velocity for SCs (−24.6%±0.9%) was significantly greater than for QCs (−21.5%±0.8%, P <0.05, t -test with Bonferroni correction for multiple testing). This difference in axonal conductive properties provides an additional line of evidence that QCs and SCs likely represent distinct classes of polymodal afferents. 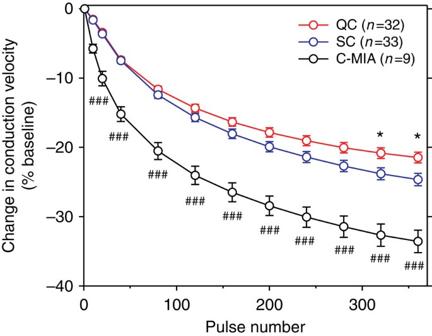Figure 3: SC afferents exhibit greater activity-dependent slowing of conduction than QC afferents. The overall decrease in conduction velocity induced by suprathreshold electrical stimulation (2 Hz for 3 min) at the receptive field differed significantly between fibre classes (F(2,73)=29.7,P<0.001). In addition, slowing over the course of the stimulation differed significantly between fibre classes (mixed model analysis of variance with pulse number and fibre class as factors (F(20,730)=9.26,P<0.001)). SC afferent slowed significantly more than QC fibres (*P<0.05,t-test with Bonferroni correction for multiple testing). C-MIAs slowed significantly more than QC- and SC-afferent fibres (###P<0.001;t-test, with Bonferroni correction for multiple testing). Error bars indicate s.e.m. Data are from pigtail and cynomolgus monkeys. Figure 3: SC afferents exhibit greater activity-dependent slowing of conduction than QC afferents. The overall decrease in conduction velocity induced by suprathreshold electrical stimulation (2 Hz for 3 min) at the receptive field differed significantly between fibre classes (F (2,73) =29.7, P <0.001). In addition, slowing over the course of the stimulation differed significantly between fibre classes (mixed model analysis of variance with pulse number and fibre class as factors (F (20,730) =9.26, P <0.001)). SC afferent slowed significantly more than QC fibres (* P <0.05, t -test with Bonferroni correction for multiple testing). C-MIAs slowed significantly more than QC- and SC-afferent fibres (### P <0.001; t -test, with Bonferroni correction for multiple testing). Error bars indicate s.e.m. Data are from pigtail and cynomolgus monkeys. Full size image QCs and SCs differ in responses to punctate chemical stimuli We previously found that cowhage spicules, which cause the sensations of itch, pricking and burning, activate QCs more vigorously than SCs ( Table 1 ). In contrast, both fibre populations were unresponsive to the intradermal injection of capsaicin [8] . In psychophysical studies, intradermal insertion of heat-inactivated spicules coated with histamine or capsaicin produced pruriceptive and nociceptive sensations similar to those evoked by active cowhage spicules [24] . Hence, active cowhage and coated spicules may activate the same set of primary afferents (that is, mechanosensitive nociceptive afferents). To test this hypothesis directly, we applied histamine- or capsaicin-coated spicules to the RFs of QCs and SCs. Whereas inactive, non-coated spicules only activated afferents during the insertion of the spicules, activity induced by spicules coated with histamine or capsaicin outlasted the application period ( Supplementary Fig. 6 ). Of the afferents tested with all three spicule preparations (inactive, histamine, capsaicin), 14/15 QCs responded to histamine and all responded to capsaicin. Of the 15 SCs tested with all three stimuli, 12 were responsive to histamine but only one responded to capsaicin-coated spicules. The incidence of capsaicin response differed significantly between QCs and SCs ( χ 2 (1) =26.65, P <0.001). The duration ( Supplementary Fig. 6 ) and magnitude ( Fig. 4a ) of the response to both histamine- and capsaicin-coated spicules were greater in QCs than in SCs. These findings demonstrate that QC afferents are capsaicin sensitive. The larger responses of QCs to superficially applied histamine and capsaicin are consistent with the notion that QC endings are located more superficially than those of SCs. 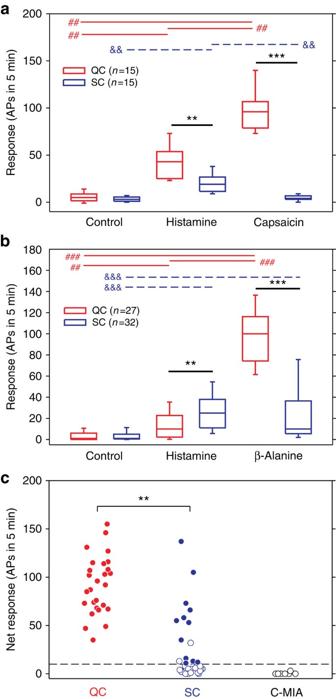Figure 4: QC and SC fibres differ in their responses to chemical stimuli. (a) QC afferents responded more vigorously than SC afferents to heat-inactivated cowhage spicules coated either with histamine (10 mg ml−1) or capsaicin (200 mg ml−1) that were inserted into the superficial layers of the skin. For each fibre class, a Friedman analysis of variance (ANOVA) was performed (QC:χ2(15,2)=26.1,P<0.001; SC:χ2(15,2)=25.0,P<0.001). Pairwise comparisons of responses to different chemical stimuli within each fibre class were then performed using Wilcoxon matched pairs test (## and &&P<0.01, with Bonferroni correction for multiple testing), comparisons across different stimuli are indicated by red and blue lines for QC and SC fibres, respectively. Responses of QC and SC fibres were compared with Mann–WhitneyU-test (**P<0.01, ***P<0.001) and comparisons are indicated by grey bars. Medians are indicated by horizontal lines, boxes represent 25th and 75th percentiles, and whiskers represent 10th and 90th percentiles. (b) Responses to intradermal injection of β-alanine (90 μg per 10 μl) were significantly greater in QC than in SC afferents (***P<0.001, Mann–WhitneyU-test). For each fibre class, a Friedman ANOVA was performed (QC:χ2(27,2)=47.4,P<0.001; SC:χ2(32,2)=33.5,P<0.001). Pairwise comparisons within each fibre class were then conducted using Wilcoxon matched pairs test (### and &&&P<0.001; ## and &&P<0.01, with Bonferroni correction for multiple testing). Responses between QC and SC classes were compared with Mann–WhitneyU-test (**P<0.01, ***P<0.001). Data representation is identical toa. (c) All 27 QC fibres responded to β-alanine, but only 12/32 SC fibres were responsive (χ2(1)=23.65,P<0.001,χ2test), and none of the MIAs responded. Net responses to β-alanine were significantly larger in responsive QC than responsive SC fibres (**P<0.01, Mann–WhitneyU-test). Open symbols correspond to fibres that did not fulfil response criteria. Dashed line indicates net response of 10 APs in 5 min. Data inaare from cynomolgus monkeys only. Data inbandcare from cynomolgus and pigtail monkeys. Figure 4: QC and SC fibres differ in their responses to chemical stimuli. ( a ) QC afferents responded more vigorously than SC afferents to heat-inactivated cowhage spicules coated either with histamine (10 mg ml −1 ) or capsaicin (200 mg ml −1 ) that were inserted into the superficial layers of the skin. For each fibre class, a Friedman analysis of variance (ANOVA) was performed (QC: χ 2 (15,2) =26.1, P <0.001; SC: χ 2 (15,2) =25.0, P <0.001). Pairwise comparisons of responses to different chemical stimuli within each fibre class were then performed using Wilcoxon matched pairs test (## and && P <0.01, with Bonferroni correction for multiple testing), comparisons across different stimuli are indicated by red and blue lines for QC and SC fibres, respectively. Responses of QC and SC fibres were compared with Mann–Whitney U- test (** P <0.01, *** P <0.001) and comparisons are indicated by grey bars. Medians are indicated by horizontal lines, boxes represent 25th and 75th percentiles, and whiskers represent 10th and 90th percentiles. ( b ) Responses to intradermal injection of β-alanine (90 μg per 10 μl) were significantly greater in QC than in SC afferents (*** P <0.001, Mann–Whitney U- test). For each fibre class, a Friedman ANOVA was performed (QC: χ 2 (27,2) =47.4, P <0.001; SC: χ 2 (32,2) =33.5, P <0.001). Pairwise comparisons within each fibre class were then conducted using Wilcoxon matched pairs test (### and &&& P <0.001; ## and && P <0.01, with Bonferroni correction for multiple testing). Responses between QC and SC classes were compared with Mann–Whitney U- test (** P <0.01, *** P <0.001). Data representation is identical to a . ( c ) All 27 QC fibres responded to β-alanine, but only 12/32 SC fibres were responsive ( χ 2 (1) =23.65, P <0.001, χ 2 test), and none of the MIAs responded. Net responses to β-alanine were significantly larger in responsive QC than responsive SC fibres (** P <0.01, Mann–Whitney U- test). Open symbols correspond to fibres that did not fulfil response criteria. Dashed line indicates net response of 10 APs in 5 min. Data in a are from cynomolgus monkeys only. Data in b and c are from cynomolgus and pigtail monkeys. Full size image β-alanine preferentially activates QC fibres In mice, about half of cutaneous unmyelinated afferents expresses MrgprD. β-alanine acts as a ligand at MrgprD [16] , [25] and activates murine non-peptidergic nociceptive afferents [16] , [26] . Intradermal β-alanine injections in humans produce the sensations of itch, pricking and burning in the absence of a flare response, suggesting that the associated itch is mediated through non-histaminergic mechanisms [16] . To investigate whether QC or SC afferents respond to β-alanine, we injected the RF with β-alanine with a dose (90 μg per 10 μl, 100 mM) that was recently used in humans [16] . QCs typically exhibited a prolonged, vigorous response to β-alanine, whereas SCs either did not respond or exhibited a comparatively weak response ( Supplementary Fig. 7 ). Consequently, the median response ( Fig. 4b ) was significantly larger in QCs than in SCs. Significantly more QCs responded to β-alanine than SCs ( Table 1 ). Of the 12 responsive SCs, only 8 responded robustly. When the analysis was restricted to β-alanine-responsive SC fibres (solid circles in Fig. 4c ), the mean net response in QCs (96.2±5.8 APs per 5 min) was still significantly larger than in these SCs (52.8±11.4 APs per 5 min, P <0.001, t -test). Based on these findings, we conclude that β-alanine preferentially activates QCs. In contrast to the finding that histamine-coated spicules produced a greater response in QCs than SCs ( Fig. 4a ), intradermal injection of histamine induced a significantly larger response in SCs ( Fig. 4b , P <0.01, Mann–Whitney U -test). However, consistent with previous findings [8] , the average net responses were not different when only histamine responsive afferents were included in the analysis (QC: 27.3±5.5 APs per 5 min versus SC: 34.5±4.5 APs per 5 min). C-MIAs respond differentially to histamine and capsaicin As C-MIAs respond vigorously to histamine and capsaicin [11] , [22] , they have been proposed to mediate both histamine-induced itch and capsaicin-induced pain. It is unclear how these two distinct sensations might be mediated through the same afferents. To address this issue, we recorded action-potential activity in C-MIAs and tested the responsiveness to intradermal injection of β-alanine (90 μg per 10 μl), histamine and capsaicin (10 μg in 10 μl each). By definition, C-MIAs had mechanical thresholds above 6 bar (8 g). Seven of the 13 C-MIAs tested were responsive to the 49 °C stimulus, and therefore represent C-heat nociceptors. Four of these showed a QC-type heat response. The mean conduction velocity of C-MIAs (0.58±0.05 m s −1 ) was significantly lower than in CMHs (0.87±0.01 m s −1 , P <0.0001, t -test). C-MIAs exhibited a progressive decrease in conduction velocity during repetitive electrical stimulation at 2 Hz ( Fig. 3 ). At the end of the stimulation, the conduction velocity decreased significantly more in C-MIAs (−34%±2%) than in SCs and QCs ( P <0.001, t -test with Bonferroni correction for multiple testing). None of the seven C-MIAs injected with β-alanine responded ( Fig. 4c ). Intradermal histamine injection produced a waxing and waning response in C-MIAs ( Supplementary Fig. 8A ). Although the overall incidence of histamine sensitivity in C-MIAs (10/13) did not differ from CMHs (33/59), the evoked net response in C-MIAs was greater ( Fig. 5a ). The median net response of histamine-sensitive C-MIAs (64.5 action potential) was greater than in histamine-sensitive CMHs (30.0 APs, P <0.05, Mann–Whitney U -test). Notably, four C-MIAs had responses greater than 150 APs per 5 min compared with none of the responsive CMHs ( P <0.01, χ 2 test, Fig. 5a ). Histamine-induced responses were long lasting with a median duration of 19.6 min (range: 2.2–20 min). 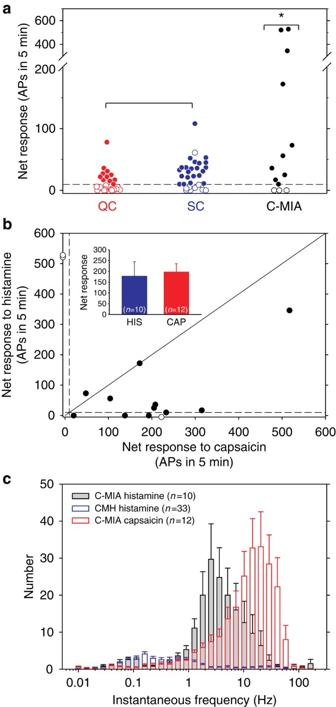Figure 5: C-MIAs are vigorously activated by histamine and capsaicin. (a) Intradermal injection of histamine produced a significantly greater net response in C-MIAs than in CMHs (*P<0.05, Mann–WhitneyU-test). Dashed line indicates net response of 10 APs in 5 min. (b) In C-MIAs tested with both histamine and capsaicin (filled circles,n=11), capsaicin responses were larger than the responses to histamine. Open circles indicate C-MIAs only tested with one agent. Inset: When only fibres that fulfil the response criteria were included, the average histamine- and capsaicin-evoked response did not differ. (c) Histograms of instantaneous frequencies of histamine responses in CMHs (blue columns) and C-MIAs (grey columns) and capsaicin responses in C-MIAs (red columns). All trials resulting in a response were included in the analysis. Bins are in log increments (factor √2). Error bars indicate s.e.m. Data are from cynomolgus and pigtail monkeys. Figure 5: C-MIAs are vigorously activated by histamine and capsaicin. ( a ) Intradermal injection of histamine produced a significantly greater net response in C-MIAs than in CMHs (* P <0.05, Mann–Whitney U- test). Dashed line indicates net response of 10 APs in 5 min. ( b ) In C-MIAs tested with both histamine and capsaicin (filled circles, n =11), capsaicin responses were larger than the responses to histamine. Open circles indicate C-MIAs only tested with one agent. Inset: When only fibres that fulfil the response criteria were included, the average histamine- and capsaicin-evoked response did not differ. ( c ) Histograms of instantaneous frequencies of histamine responses in CMHs (blue columns) and C-MIAs (grey columns) and capsaicin responses in C-MIAs (red columns). All trials resulting in a response were included in the analysis. Bins are in log increments (factor √2). Error bars indicate s.e.m. Data are from cynomolgus and pigtail monkeys. Full size image Intradermal capsaicin injection produced high-frequency bursting discharge in C-MIAs ( Supplementary Fig. 8A ). Capsaicin activated heat-sensitive and heat-insensitive C-MIAs and the response did not significantly differ between these groups. The incidence of afferents responding to intradermal capsaicin injection was significantly greater in C-MIAs (12/12) than that previously shown by us [8] for CMHs (3/25, P <0.001, χ 2 test). Most of the C-MIAs (10/12), but none of the three responsive CMHs, responded with more than 100 APs per 5 min ( P <0.001, χ 2 test; Fig. 5b ). Of the three responsive CMHs, two barely fulfilled the response criteria. The CMH with the highest response produced 80 APs in 5 min compared with 529 APs per 5 min in the largest C-MIA responder. Similar to histamine, capsaicin induced lasting responses in C-MIAs (median duration: 10.2 min; range: 0.46–19.9 min) with four responding for more than 18 min. The average responses of C-MIAs to histamine and capsaicin were not different ( Fig. 5b insert). However, for the 11 C-MIAs tested with both (filled symbols in Fig. 5b ), three fibres did not respond to histamine, and the capsaicin-evoked net response (195.7±40.9 APs per 5 min) was significantly greater than that produced by histamine (66.8±31.8 APs per 5 min, P <0.01, Wilcoxon matched pairs). This apparent discrepancy is due to the fact that the two highest histamine responders were not tested with capsaicin (open symbols, Fig. 5b ) Although the total responses to histamine (172 APs) and capsaicin (182 APs) were similar in the example C-MIA, the temporal patterns of discharge were quite different ( Supplementary Fig. 8 ); histamine produced a periodic waxing and waning response whereas capsaicin induced high-frequency bursts. To investigate discharge patterns across the population of CMHs and C-MIAs, we generated instantaneous frequency histograms for the histamine and capsaicin responses. All fibres with a positive response were included in the analysis. For histamine-induced activity, the instantaneous frequency distribution in C-MIAs was significantly different from CMHs ( Fig. 5c , Kolmogorov–Smirnov test for two samples, P <0.001). The median discharge frequency in C-MIAs (2.7 Hz) was more than seven times the median discharge in CMHs (0.37 Hz). For C-MIAs, the instantaneous frequency distribution for the histamine response was significantly different from that to capsaicin ( Fig. 5c , P <0.001, Kolmogorov–Smirnov test for two samples). The median discharge frequency induced by capsaicin (12 Hz) was more than four times that induced by histamine (2.7 Hz). β-alanine and histamine activate different DRG neurons Functional investigation of calcium imaging on cultured primate DRG neurons shows that β-alanine responsive neurons are distinct from the histamine-responsive population. Using concentrations that have previously been used in mice DRG neurons [16] , [27] , we tested 484 cells from three monkeys in the order of β-alanine (1 mM, 89 μg ml −1 ), histamine (100 μM, 11 μg ml −1 ) and capsaicin (5 μM, 1.5 μg ml −1 ), each separated with at least a 3-minute wash for the cells to recover ( Fig. 6a,b , Supplementary Fig. 9 ). Eight percent of the cells were β-alanine responsive (39/484), 9% were histamine responsive (43/484) and 26.9% (130/484) were capsaicin responsive. Less than 1% of the cells responded to both histamine and β-alanine (4/484). Moreover, 64% of β-alanine responsive cells were capsaicin responsive (25/39) ( Fig. 6c ). Interestingly, 14% of the histamine-responsive cells (6/43) responded only to histamine. 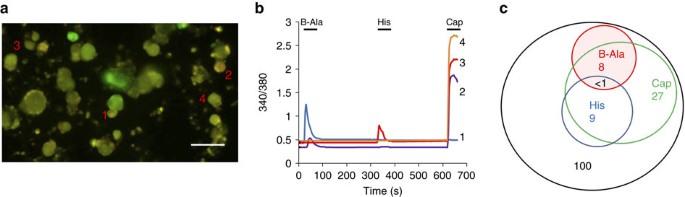Figure 6: Histamine and β-alanine activate different populations of DRG neurons. (a) Specimen fluorescent picture of cultured DRG neurons investigated in calcium imaging studies. The intracellular calcium levels of the neurons numbered are shown in the traces inb. (Scale bar, 100 μm). (b) Traces of intracellular calcium responses from representative cells ina. Cells were tested with β-alanine (1 mM, 60 s), histamine (100 μM, 40 s) and capsaicin (5 μM) with at least a 3-min washout period between applications. Cells with an increase above 20% in the 340/380 ratio were classified as responders. Cell #1 and #2 are responsive to β-alanine but not histamine. In contrast, cell #3 is responsive to histamine but not β-alanine, whereas cell #4 only responds to capsaicin. (c) Venn diagram shows the incidence of response (percent) to different reagents. β-alanine responsive cells are separate from histamine-responsive cells. The majority of the β-alanine and histamine responsive cells also respond to capsaicin. A total of 484 cells from three monkeys were analysed: 8% responded to β-alanine, 9% to histamine and 27% to capsaicin. Less than 1% of the cells responded to both β-alanine and histamine, suggesting that β-alanine and histamine-responsive cells are separate subpopulations in DRG. Data are from cynomolgus monkeys only. Figure 6: Histamine and β-alanine activate different populations of DRG neurons. ( a ) Specimen fluorescent picture of cultured DRG neurons investigated in calcium imaging studies. The intracellular calcium levels of the neurons numbered are shown in the traces in b . (Scale bar, 100 μm). ( b ) Traces of intracellular calcium responses from representative cells in a . Cells were tested with β-alanine (1 mM, 60 s), histamine (100 μM, 40 s) and capsaicin (5 μM) with at least a 3-min washout period between applications. Cells with an increase above 20% in the 340/380 ratio were classified as responders. Cell #1 and #2 are responsive to β-alanine but not histamine. In contrast, cell #3 is responsive to histamine but not β-alanine, whereas cell #4 only responds to capsaicin. ( c ) Venn diagram shows the incidence of response (percent) to different reagents. β-alanine responsive cells are separate from histamine-responsive cells. The majority of the β-alanine and histamine responsive cells also respond to capsaicin. A total of 484 cells from three monkeys were analysed: 8% responded to β-alanine, 9% to histamine and 27% to capsaicin. Less than 1% of the cells responded to both β-alanine and histamine, suggesting that β-alanine and histamine-responsive cells are separate subpopulations in DRG. Data are from cynomolgus monkeys only. Full size image There is considerable functional, anatomical and developmental heterogeneity among nociceptive afferent neurons [28] , [29] , [30] . Much progress has been made in mice to differentiate the role of different subclasses of DRG neurons in behaviour [16] , [17] , [18] , [20] , [31] , [32] . How these findings translate to primates is currently unclear, as many of the techniques used in mice cannot be employed in primates. Using teased-fibre techniques to record single-unit activity from primate cutaneous unmyelinated afferents, we provide several lines of evidence that two functionally distinct classes can be differentiated among mechanoheat sensitive C fibres. These classes differed significantly in 22 of 25 physiological measures of responsiveness. We furthermore provide evidence for a peripheral coding of pruriceptive and algogenic stimuli in C-MIAs. Mechanosensitive C-fibre nociceptors exhibited either a quick (QC) or a slow (SC) response to a stepped heat stimulus. As QCs and SCs could be differentiated in two primate species, such differentiation likely also exists in other species, including humans. We hypothesized previously that the different heat responses are explained by receptive terminals being located at different depths within the skin. Here we tested the alternative hypothesis that QCs and SCs represent two distinct populations which respond differentially to a range of different stimuli. QCs were more sensitive to mechanical and heat stimuli than SCs, which is consistent with the interpretation that the receptive terminals of QCs are situated more superficially within the skin than SC terminals. However, depth alone cannot explain that SCs sensitized more to heat than QCs following a mild burn injury. Particularly, QCs and SCs exhibited different temperature-dependent heat sensitization, and QCs and SCs responded differentially to the sensitizing stimulus itself ( Fig. 2d ). These findings indicate that QCs and SCs differ in heat transduction and/or heat sensitization mechanisms. What are the mechanisms underlying the two types of heat responses? Transient receptor potential vanilloid 1 (TRPV1) [33] , transient receptor potential melastatin-3 [34] and anoctamin 1 [35] have been identified as transduction proteins for noxious heat. Transient receptor potential melastatin-3 and anoctamin 1 are co-expressed with TRPV1 in nociceptive neurons [34] , [35] . The marked QC/SC difference in heat sensitivity may be due to a differential expression of these transduction channels. The heat response may also depend on mediators (for example, ATP) released from non-neuronal skin cells (for example, keratinocytes) upon heat stimulation. Such a mechanism has previously been proposed for the detection of ‘warm’ temperatures [36] , but it is unclear if it plays a role in the detection of noxious heat. Finally, the ion channels expressed at the spike initiation site may differ and contribute, for example, to the differences in peak discharge frequency and adaptation rates to a ‘stepped’ heat stimulus. We do not know what explains the marked QC/SC difference in heat sensitization. Multiple inflammatory mediators can sensitize nociceptive afferents to heat (for example, bradykinin, prostaglandins), and, in addition to differences in heat transduction mechanisms, QCs and SCs may differ in their susceptibility to the action of these mediators. Activity-dependent slowing of conduction velocity during repetitive electrical stimulation differs significantly between unmyelinated fibres of different receptive properties [37] , [38] , [39] . We found that activity-dependent slowing of conduction velocity in QCs was significantly less than in SCs. Although the difference was small, it provides additional evidence for an inherent difference between these C-fibre classes that is independent of heat transduction mechanisms and skin depth. The inactivation of sodium channels likely contributes to this phenomenon [40] . The observed difference may indicate a differential expression of sodium channels along the axonal membrane or, alternatively, differences in Na–K–ATPase activity that retrieves channels from the inactivated state. Heat-inactivated cowhage spicules coated with histamine or capsaicin have been used to apply chemical stimuli, in a punctate manner, to human skin to investigate the neuronal mechanisms underlying itch sensation [24] , [41] . In contrast to intradermal capsaicin injection, which evokes intense dose-dependent pain [42] , superficial topical application [43] or punctate application via inactivated cowhage spicules causes itch that is accompanied by nociceptive sensations similar to the sensations caused by native cowhage spicules [24] . In mice, most polymodal C-fibres were activated by capsaicin-coated spicules, and a subset of these were also activated by histamine-coated or active cowhage spicules [44] . Both QCs and SCs responded to histamine-coated spicules, but responses in QCs were significantly larger than in SCs. Similarly, active cowhage spicules induced significantly larger activity in QCs than SCs [8] . In contrast to findings in mice [44] , capsaicin-coated spicules produced a strong and lasting excitation only in a functionally distinct subset of polymodal CMH, that is, QCs but not SCs. A more superficial location of receptive terminals in the skin could, at least in part, account for the significantly larger activation of the QCs than SCs. However, other factors including differences in expression of membrane receptors and ion channels may contribute. The capsaicin responses in QCs are unlikely due to a nonspecific effect as SCs are unresponsive to the same stimulus. A lack of response to capsaicin-coated spicules has also been observed in mechanosensitive but heat-insensitive murine C-fibre neurons [44] . Thus, the response to capsaicin-coated spicules appears to be linked to heat sensitivity although not all heat-sensitive afferents (for example, SCs) are responsive. The vigorous excitation in QCs by capsaicin-coated spicules contrasts with our own and other previous studies that observed only a short lasting excitation in the majority of polymodal nociceptors following intradermal capsaicin injection [8] , [10] , [11] , [45] . However, topical application of capsaicin solution has been reported to activate polymodal nociceptors in primate [10] . Together, these findings indicate that the psychophysical and electrophysiological capsaicin effects vary with application mode. One possible explanation for the difference between the responses to superficial application via coated spicules and intradermal injection is that with injection, the peripheral terminals and also the parent axon are ‘bathed’ in capsaicin. As TRPV1 is expressed along the axonal membrane of unmyelinated fibres [46] , capsaicin may produce a conduction block by inhibiting sodium channel function through TRPV1-dependent [47] and TRPV1-independent mechanisms [48] , [49] . That polymodal nociceptors become desensitized following intradermal injection of capsaicin but not following application with coated spicules is consistent with such an interpretation [8] , [10] , [11] . QCs likely contribute to itch and nociceptive sensations induced by capsaicin-coated spicules in humans [24] , [41] , although mechanically insensitive afferents may also contribute, as capsaicin-coated spicules produce a flare reaction in human skin [41] . As heat hyperalgesia depends on TRPV1 expression [50] , [51] , the lack of response in SCs to capsaicin-coated spicules appears in contrast to the marked heat sensitization in these afferents. Our results suggest that SCs express only low levels of TRPV1 on their axonal membranes, or alternatively, that TRPV1 function is inhibited in SCs under normal physiological conditions. During inflammation, such as following a mild burn injury, however, TRPV1 becomes sensitized by released inflammatory mediators and trafficking of TRPV1 to the cell membrane is increased (for review see ref. 52 ). Regardless of application mode, histamine elicited a relatively weak response in CMHs (compared with C-MIAs). This small discharge may not significantly contribute to histamine itch in primate, consistent with a recent psychophysical study in humans showing that C-MIA alone are sufficient to mediate histamine itch [53] . The low histamine-induced activity in CMHs may furthermore be too small to generate a detectable signal in calcium imaging studies. C-MIAs respond vigorously to intradermal injection of histamine and capsaicin as has been observed previously in microneurography studies in humans [11] , [22] . In contrast to these studies that rely on marking techniques to quantify indirectly neuronal responses, we are able to directly compare histamine- and capsaicin-induced action potential discharges. Some fibres tested with both substances only responded to capsaicin. These C-MIAs likely represent nociceptive-specific afferents unresponsive to pruriceptive stimuli. In histamine-responsive C-MIAs, capsaicin produced a significantly larger response than histamine (see Fig. 5c ). Therefore, these afferents are pruriceptive nociceptive afferents with a selective response to algogenic stimuli. When compared across all C-MIAs tested with and responsive to histamine and capsaicin, the evoked response did not differ between capsaicin and histamine (see inset Fig. 5b ). However, the discharge patterns were quite different; capsaicin induced bursts of activity that contained high instantaneous frequency discharges, whereas histamine induced sustained low instantaneous frequency discharges. These observations provide a potential mechanism by which C-MIAs could encode for both capsaicin pain and histamine itch. Our findings do not rule out the existence of histamine-specific C-MIAs (two C-MIAs with the highest response to histamine were not tested with capsaicin) that would constitute a labelled line for histamine itch. Indeed, our calcium imaging studies revealed some cells with a response to histamine only. However, histamine itch can be abolished in humans by capsaicin desensitization of the skin [54] , [55] and histamine itch is mediated through TRPV1 [56] , [57] . Furthermore, histamine itch is abolished when TRPV1 expressing axons have been silenced by co-application of capsaicin and QX-314 [58] . Therefore, it is unlikely that a capsaicin-insensitive, histamine-sensitive labelled line for itch exists. Our findings instead suggest that histamine itch is encoded by low level (~\n2 Hz) neuronal activity in pruriceptive, nociceptive C-MIAs in the absence of activity in nociceptive-specific C-MIAs. Together with capsaicin sensitive Aδ-MIAs [59] , capsaicin-sensitive C-MIAs likely encode capsaicin pain. It is likely that DRG cells with the greatest calcium signal in response to histamine and capsaicin belong to the C-MIA class. In calcium imaging studies, the percentage of neurons being sensitive to a chemical stimulus was lower than in teased fibre experiments. This discrepancy is not surprising as DRGs contain the soma of visceral neurons and those innervating muscle, joints and skin. In contrast, peripheral nerve recordings were performed on cutaneous afferents. C-MIAs did not respond to β-alanine in peripheral nerve recordings. This is consistent with results from calcium imaging studies showing little overlap between neuronal populations responding to histamine and β-alanine. Cross-desensitization/sensitization of β-alanine and histamine likely contributed little, if any, to our results in calcium imaging studies as evidence from mice demonstrates that β-alanine- and histamine-responding sensory neurons are separate populations [16] , [32] . Intradermal injection of β-alanine activated all QCs but only 40% of SCs, and the activity in QCs was twice that of responsive SCs. All afferents responsive to β-alanine were responsive to noxious heat stimuli, a finding similar to those reported in mice [16] , [26] . QCs were also activated by capsaicin-coated spicules, which is consistent with our observations from calcium imaging studies in which β-alanine-responsive neurons were also activated by capsaicin. Intradermal β-alanine injection does not produce a flare response [16] , and as QCs are activated by capsaicin-coated cowhage spicules, and cowhage-induced itch is abolished in capsaicin desensitized skin [12] , QCs likely represent non-peptidergic, TRPV1- and MrgprD-expressing neurons. Although, we cannot exclude the possibility that β-alanine may excite nociceptive afferents in primate through a receptor other than MrgprD, this appears unlikely, as the effects of β-alanine were lost in MrgprD −/− mice [16] . For SCs, such classification is less straightforward, as 40% responded to β-alanine and the vast majority did not respond to capsaicin-coated cowhage spicules. However, SCs showed marked sensitization to heat stimuli, a function thought to depend on the expression of TRPV1 [50] , [51] . Based on findings in mice [16] showing that β-alanine only excites mechanoheat-sensitive MrgprD neurons, we suggest that the remaining 60% of SCs not responding to β-alanine represent MrgprD negative, peptidergic afferents. The QC/SC difference in heat and mechanical thresholds and the difference in their responses to superficially applied chemical stimuli may be, at least in part, due to the difference in epidermal layers targeted by non-peptidergic and peptidergic afferents [32] , [60] . Animals All experiments were performed in accordance with the Animal Welfare Act regulations and the USPHS Policy on Humane Care and Use of Laboratory Animals and approved by the Johns Hopkins University Animal Care and Use Committee. Adult (3–10 years of age), male cynomolgus ( Macaca fascicularis , n =13) and pigtail monkeys ( Macaca nemestrina , n =6) were used. Animal preparation Animals were sedated by intramuscular ketamine (Ketaject, Phoenix, St. Joseph, MO; 12 mg kg −1 ). A pentobarbital bolus (6 mg kg −1 , Nembutal, Ovation Pharmaceuticals, Deerfield, IL) was administered via an intravenous catheter to induce anaesthesia. A continuous infusion of pentobarbital at 4–6 mg kg −1 h −1 was given to maintain anaesthesia. Core temperature was maintained near 38 °C using feedback-controlled warm-water heating pads, and an intravenous drip of 5% dextrose was continuously given for hydration. Heart rate was monitored and depth of anaesthesia was adjusted, if tachycardia occurred in response to noxious stimuli. Following intubation, paralysis was induced with pancuronium bromide (SICOR Pharmaceuticals, Irvine, CA; 0.1 mg kg −1 every 2 h), and animals were ventilated to maintain a pCO2 of 35–40 mm Hg. A prophylactic antibacterial agent, Cefazolin (West-Ward Pharmaceutical, Eatontown, NJ; 20 mg kg −1 h −1 ), was administered. At the end of the experiment and on the following postoperative day, animals received buprenorphine (Buprenex Injectable, Reckitt Benckiser Pharmaceuticals, Richmond, VA; 0.15 mg per injection). Recordings were made from multiple cutaneous nerves in a given animal with experiments being separated by at least 2 weeks. After all peripheral nerve recordings were completed, three animals were euthanized for harvesting DRG tissues for calcium imaging experiments. Using aseptic techniques, nerves were dissected under a microscope, and a standard teased-fibre technique [8] , [61] was used to record neuronal activity in single afferent fibres. Peripheral nerves innervating the hairy skin were used for recordings (saphenous, superficial peroneal, sural, superficial radial and medial antebrachial cutaneous nerves). A bundle of the dissected nerve was cut proximally and split into smaller strands on a dissecting platform that also served as a reference electrode and supported the nerve trunk. The strands were placed on the recording electrode, situated in the near vicinity of the splitting platform. About 4 cm distal to the recording electrode, a stimulating electrode was positioned on the nerve trunk to identify slowly conducting unmyelinated nerve fibres (conduction velocity 0.5–2 m s −1 ). Data recording APs were filtered, amplified and digitized (Digital Acquisition Processor board, Microstar Laboratories, Bellevue, WA) for storage on a personal computer. The interface was operated using DAPSYS software (v.7; Brian Turnquist, see www.dapsys.net ) for Windows. The software allowed for action potential discrimination, action potential timing, timing of events that occurred during the recordings (for example, start baseline, stop baseline, stimulus applications, injections), and control of the laser stimulus parameters. Initial characterization of afferent nerve fibres and QC/SC classification Gentle squeeze stimuli were applied to the skin to locate RF of unmyelinated afferents. The mechanosensitive RF was then mapped with an 8.9 bar (15 g) von Frey hair. Mechanosensitive spots within this RF were located with a suprathreshold von Frey hair. The spot most sensitive to a slightly suprathreshold von Frey hair was used to determine the mechanical threshold of the unit under study. After a 2-min rest, a series of von Frey hairs of increasing intensity were applied to this spot and the smallest von Frey hair that activated the unit in two out of four applications (>3 s between stimuli) was regarded as threshold. An epoxy-coated brass rod and a refrigerated brass rod were applied to the RF to determine the sensitivity of the afferent to blunt pressure and cold. To determine the conduction velocity of the unit from the skin, transcutaneous electrical stimuli were applied through ball electrodes placed on the skin a few millimetres proximal to the mechanosensitive RF. Repetitive electrical stimuli (0.25 Hz) of increasing current (0.1–1 ms duration) were applied, and the smallest current intensity that could activate the afferent was regarded as electrical threshold. When current was increased beyond this threshold, the conduction latency decreased in discrete steps indicating the activation of faster conducting and deeper terminal branches in the skin [59] , [62] , [63] . The latency measured at the highest stimulation intensity (100 mA) was regarded as the shortest conduction latency and likely represents activation of the afferent fibre at the parent axon. Current intensity was then set to an intensity at which the afferent could be recorded with a stable conduction latency. Collision between electrical stimuli applied at the skin and at the nerve trunk electrode was then performed to determine the conduction latency of the afferent fibre from the nerve trunk. In some of the experiments, we then performed repetitive electrical stimulation to study the conductive properties (see Methods on Conduction properties for details below) of the unit under study. In a subset of afferents, we then tested the responsiveness to suprathreshold mechanical stimuli (see Methods on Suprathreshold mechanical stimulation for details below) prior to testing sensitivity to heat. The responsiveness to noxious heat was tested by applying heat stimuli using a contact-free, temperature-controlled CO 2 laser stimulator system [64] . Ten minutes after application of the test stimulus (49 °C, 3 s) to classify fibres as QC or SC, a staircase heat stimulus (baseline (36 or 38 °C) for 15 s followed by temperature steps (1 °C, 1 s) from 37 or 39–49 °C) was applied to determine heat threshold (lowest temperature at which the first action potential could be recorded) and to evaluate the development of the heat response with increasing temperature. The baseline temperature of 36 °C was chosen for the staircase stimulus if the fibres had responded to the 38 °C baseline temperature of the 49 °C, 3-s stimulus. The sum of APs to the staircase was calculated as the total response. In experiments investigating the effects of a mild burn injury, however, the baseline of the staircase heat stimulus was set at 36 °C and temperature steps ranged from 37–49 °C (see Methods on Heat Sensitization for more details below). Ten minutes following this initial battery of tests to characterize the afferent fibre, the specific protocols described below were executed in different subsets of fibres. For the classification of an afferent as QC/SC, the time of peak instantaneous discharge in response to a 49 °C, 3-s heat stimulus was used. Peak instantaneous discharge and time of peak instantaneous discharge (relative to stimulus onset) were determined after 3-point median smoothing was applied to the raw instantaneous discharge frequencies of the APs (except the first and last action potential) recorded during this heat stimulus. This procedure lessened the influence of a single-action potential on the classification, thereby minimizing the potential for misclassification. Median smoothing was performed in Microsoft Excel (2003) after raw data had been exported from DAPSYS. Suprathreshold mechanical stimulation Responses to suprathreshold mechanical stimulation were tested prior to applying heat stimuli in a subset of afferents. Fibres were tested, at the most sensitive spot in the RF, with three von Frey hairs exerting different mechanical pressure (4.1, 6 and 8.9 bars). With the aid of a microscope, each von Frey hair was applied at that spot for 3 s and tested three times at an interstimulus interval of 20 s. After a 2-min rest period, the next higher von Frey hair was applied employing an identical protocol. Stimuli were applied with all audio equipment switched off so that the experimenter applying the von Frey hair was unaware of the induced responses. For analysis, the median response of the three applications of a given von Frey hair was used. Cold stimulation Responsiveness to cold stimuli was tested by applying a chilled (4 °C) brass probe (19 mm diameter) to the RF for 20 s. As a control, an identical brass probe of room temperature with a plastic-coated end was applied to the RF. An afferent fibre was classified as ‘cold’ responsive if the response to cold probe was at least 10 APs greater than the response to the control probe. Punctate chemical stimulation To test for responsiveness to punctate chemical stimulation, heat-inactivated cowhage spicules were coated with histamine or capsaicin [24] , [41] , [44] . Briefly, inactive spicules were soaked in histamine solution (10 mg ml −1 prepared in distilled water) or capsaicin solution (200 mg ml −1 prepared in 80% ethanol) for 12 h, dried and then loaded onto the tips of cotton swab applicators that had been slightly coated with a layer of compound Q (Apiezon, Manchester, UK). To establish a ‘control’ response in a given afferent, we first tested the response to inactive cowhage spicules (single trial), followed by three trials each for histamine- and capsaicin-coated spicules. The trial with the maximum response was used for subsequent analysis. A single trial for inactive spicules was regarded as sufficient, as these produced only a weak activation in unmyelinated afferents in a previous study [8] . Following a 1-min period in which baseline activity was recorded, spicules were applied, during a 15-s period, to the receptive field by pressing the applicators against the skin resulting in an average of 16 spicules (range: 3–35) being inserted into the epidermis. Neuronal activity was then recorded for a minimum of 5 min up to a total of 20 min. Recordings were stopped after 5 min if no neuronal activity was recorded or at any time point thereafter when no neuronal activity was recorded for three consecutive minutes. After the end of a trial, spicules were picked from the skin with forceps, and the next trial was initiated after a 2-min rest period. To compare the responses induced by different chemicals, spontaneous activity encountered during the baseline was prorated and subtracted from the response observed in 5 min. From this response, the vehicle response was subtracted to calculate the net response. Afferents were considered ‘responders’, if this net response was (1) at least 10 APs, and (2) greater than the response to the control (uncoated, inactive spicules or vehicle injection). Heat sensitization After a rest period (10 min) to allow recovery from fatigue induced by the initial heat stimulus (49 °C for 3 s) used to classify an afferent as QC/SC, heat responsiveness was assessed by three consecutive heat staircase stimuli (36 °C baseline for 15 s followed by 37–49 °C in 1 °C, 1-s steps, 10 min interstimulus interval) applied to the RF. Ten minutes after the third staircase stimulus, a mild burn injury (48 °C for 120 s) was produced at the RF. In humans, such injury leads to marked heat hyperalgesia without obvious skin injury (that is, blister) [23] . To assess sensitization-induced changes in heat responses, a second block of three heat staircases was applied starting 10 min after the burn injury. For data analysis, the number of APs recorded at a given temperature was averaged for the three staircases pre- and post-burn injury. Heat threshold was defined as the lowest temperature at which an action potential was recorded without correcting for conduction latency. Conduction properties We used a stimulation paradigm (2 Hz, 3 min) that has previously been shown to differentiate functionally distinct classes of primary afferent nerve fibres in humans, rat and pig [37] , [39] , [65] . After a 2-min rest period, electrical stimuli were applied transcutaneously through ball electrodes positioned slightly proximal to the mechanosensitive RF. Current was initially set to an intensity at which a stable latency could be recorded for the afferent fibre when stimulated at a frequency of 0.25 Hz. For some afferent fibres, stimulus intensity had to be increased during to the 2 Hz stimulation, as the afferent became unresponsive to the originally chosen current intensity. For analysis, we determined for each action potential initiated during repetitive stimulation (2 Hz, 3 min), the conduction latency relative to the time of the initiating stimulus. We also determined the amount of total latency increase between the last and the first action potential initiated by 2 Hz stimulation. Conduction velocities and changes thereof were calculated by dividing the distance between stimulating and recording electrodes by the measured latencies. Intradermal injection studies Histamine dihydrochloride and β-alanine were purchased from Sigma-Aldrich (St Louis, MO). Solutions were prepared in extracellular fluid according to a previous study [41] . Afferents studied with this protocol were first injected with vehicle (extracellular fluid, 10 μl) followed by an injection of β-alanine (100 mM; 90 μg per 10 μl) and histamine (10 μg per 10 μl). For about half the fibres tested, histamine was injected prior to β-alanine. All injections were performed at the same site within the mechanosensitive RF, that is, the most sensitive spot to mechanical stimulation. After a baseline of 1 min to record spontaneous activity, histamine or β-alanine was injected and neuronal activity was recorded for a minimum of 5 min. Recordings were continued for a maximum of 20 min but could be aborted if no activity had been recorded for three consecutive minutes. Data were analysed and fibres classified as ‘responders’ as described under Punctate chemical stimulation above. Calcium imaging studies DRG from Macaca fascicularis were collected in cold DH10 medium (90% DMEM/F-12, 10% FBS, 100 U ml −1 penicillin, and 100 μg ml −1 Streptomycin, Gibco) and treated with enzyme solution containing collagenase (1.65 mg ml −1 , Worthington CLS I) and dispase (3.55 mg ml −1 , GIBCO 17105-041) at 37 °C for 1 h. After trituration and centrifugation, cells were resuspended in DH10, plated on glass coverslips coated with poly- D -lysine (0.5 mg ml −1 , Stoughton, MA) and laminin (10 μg ml −1 , Invitrogen), cultured in an incubator at 37 °C overnight. Those neurons were tested within 48 h. DRG neurons were loaded with 2 μM fura 2-acetomethoxy ester (Molecular Probes) for 30 min in the dark at room temperature. After washing, cells were imaged at 340 and 380 nm excitation to detect intracellular free calcium under fluorescent microscope (Nikon Eclipse TE2000-S) and Lambda 10B shutter (Sutter Instrument). The cells were bathed in the calcium imaging buffer (pH 7.45, 130 mM NaCl, 3 mM KCl, 2.5 mM CaCl 2 , 10 mM HEPES, 10 mM glucose, 1.2 mM NaHCO 3 , with sucrose adding up the osmolarity to 290 mOsm). The reagents and buffers were applied through gravity perfusion system at the rate of 2 ml s −1 . Images were processed and analysed with the software NIS-Elements BR 2.30 (Nikon.) A responsive cell is defined as one that has more than 20% increment in 340/380 ratio over the baseline. Statistical analysis Data were analysed using Statistica 6.1 (StatSoft, Tulsa, OK). Normally distributed data were analysed with parametric tests, otherwise non-parametric tests were used (see text for details). A P <0.05 was regarded as significant. Data are presented as mean±s.e.m. or median, 10th, 25th, 75th and 90th percentile where appropriate. How to cite this article : Wooten, M. et al. Three functionally distinct classes of C-fibre nociceptors in primates. Nat. Commun. 5:4122 doi: 10.1038/ncomms5122 (2014).